Hierarchical structural design for fracture resistance in the shell of the pteropodClio pyramidata The thecosomes are a group of planktonic pteropods with thin, 1 mm-sized aragonitic shells, which are known to possess a unique helical microstructure consisting of interlocking nanofibres. Here we investigate the detailed hierarchical structural and mechanical design of the pteropod Clio pyramidata . We quantify and elucidate the macroscopic distribution of the helical structure over the entire shell (~1 mm), the structural characteristics of the helical assembly (~10–100 μm), the anisotropic cross-sectional geometry of the fibrous building blocks (~0.5–10 μm) and the heterogeneous distribution of intracrystalline organic inclusions within individual fibres (<0.5 μm). A global fibre-like crystallographic texture is observed with local in-plane rotations. Microindentation and electron microscopy studies reveal that the helical organization of the fibrous building blocks effectively constrains mechanical damages through tortuous crack propagation. Uniaxial micropillar compression and cross-sectional transmission electron microscopy directly reveal that the interlocking fibrous building blocks further retard crack propagation at the nanometre scale. Driven by the need for new lightweight composites with improved mechanical properties and cost-effective and environmentally friendly manufacturing strategies [1] , [2] , many engineers are now turning to nature for design insight into the fabrication of damage tolerant and hierarchically ordered structural materials [3] , [4] , [5] . Biomineralized composites, such as bone, sponge spicules and mollusc shells, for example, demonstrate excellent mechanical properties, especially considering their relatively soft/weak organic and stiff/brittle ceramic constituents [6] , [7] , [8] , [9] , [10] . In addition, these biological materials often exhibit remarkable hierarchical structural complexity spanning from the nanoscale to the macroscale. Here we report a comprehensive investigation of the structure–property relationships of one such example, the multifunctional mineralized shell of the pteropod, Clio pyramidata (Linnaeus 1767), which is simultaneously mechanically robust, optically transparent and lightweight. Pteropods are a polyphyletic group of small marine planktonic gastropods consisting of two evolutionarily unrelated clades, the Thecosomata and Gymnosomata. Species from both clades are pelagic and highly transparent, and swim using wing-like flaps derived from their modified foot. In contrast to the gymnosomes that lack shells, thecosomes have thin transparent aragonitic shells exhibiting a diversity of geometries including coiled, needle-like, triangular and globose forms [11] . More than five formae (subspecies) belong to the species Clio pyramidata , each of which is characterized by its distinctive shell geometry [12] , [13] . In this work, we investigate the shell of the lanceolata form (Lesueur, 1813) as a representative member of the group. The thin transparent shell of C. pyramidata exhibits an uncoiled pyramid-like shape ( Fig. 1a,b ), with three diverging longitudinal ribs that form an anterior opening. 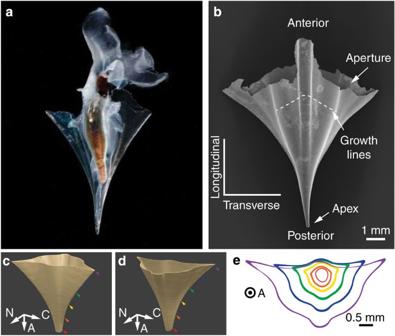Figure 1:Macroscopic geometry of theC. pyramidatashell. (a) Photograph of a liveC. pyramidata(used with permission from Dr Danté Fenolio). (b) Dorsal-viewed SEM image showing the pyramidally shaped shell. 3D reconstructions of the shell in (c) ventral and (d) dorsal views based on X-ray micro-computed tomography data. (e) Transverse cross-sections of the shell at different heights indicated by the arrows with corresponding colours incandd. A pseudo-cylindrical coordinate system is defined as following: N (normal), the surface normal direction; A (apical), the direction towards the shell’s apex; C (circumferential). Figure 1: Macroscopic geometry of the C. pyramidata shell . ( a ) Photograph of a live C. pyramidata (used with permission from Dr Danté Fenolio). ( b ) Dorsal-viewed SEM image showing the pyramidally shaped shell. 3D reconstructions of the shell in ( c ) ventral and ( d ) dorsal views based on X-ray micro-computed tomography data. ( e ) Transverse cross-sections of the shell at different heights indicated by the arrows with corresponding colours in c and d . A pseudo-cylindrical coordinate system is defined as following: N (normal), the surface normal direction; A (apical), the direction towards the shell’s apex; C (circumferential). Full size image A variety of microstructural design strategies have been reported for aragonite-based mollusc shells, among which, the damage tolerant cross-lamellar [7] , [14] and nacreous-based [15] shells have been the most extensively characterized. In contrast to a majority of other mollusc shells, those from pteropods [11] , [16] and heteropods [17] exhibit a unique helical microstructure. This helical microstructure is expected to exhibit enhanced damage tolerance, similar to recently reported structural assemblies of macroscopic topological interlocking building blocks [18] , [19] . Indeed, observations of fractured petropod shells reveal such tortuous fracture pattern; recent nanoindentation-based experiments on the petropod shell of Cavolinia uncinata also suggest that the helical assembly might result in the anisotropic mechanical properties [20] . The objectives of the present study were to investigate the full hierarchical structural characteristics of the shell from C. pyramidata at multiple length scales; to establish the correlation between the crystallographic texture and the multiscale structural features; and to investigate the multiscale mechanical behaviour in relation to its hierarchical structural design and ascertain the role of the helical microstructure in the shell’s fracture resistance. The mechanistic understanding of the enhanced fracture resistance in this complex material system holds great potential in the development of bio-inspired engineering materials with improved mechanical properties. Helical assembly Three-dimensional reconstructions of the shell from C. pyramidata based on X-ray micro-computed tomography data are shown in Fig. 1c–e and clearly illustrate the shell’s bilateral symmetry. From the posterior to the anterior region of the shell, the transverse cross-sectional geometry gradually changes from a tube-like to a triangular form ( Fig. 1e ). A pseudo-cylindrical coordinate system was used for denoting the sample orientations, where N (normal) refers to the surface normal direction, A (apical) and C (circumferential) refer to the longitudinal and transverse directions in the surface tangent plane, respectively. A fractured surface of the C. pyramidata shell reveals a microstructure composed of densely packed curved fibrous building blocks ( Fig. 2a–c ), similar to other pteropod and heteropod shells [11] , [16] , [17] , [20] . Following previous studies [11] , [16] , [17] , [20] , it is proposed that the curved fibres form a helical assembly in which the helical axis is normal to the shell surface (along N, Fig. 2d ); however, no direct evidence indicates that the fibrous building blocks themselves are complete helices through the shell thickness, a topic which will be discussed in detail below. The radius of the helical assembly, R , was estimated to be 10–15 μm from the bottom-viewed fractured surface as shown in Fig. 2b,d ). The helical assembly of the rotating building blocks is further illustrated in the three-dimensional (3D) reconstruction of the fractured surface, derived from stereo image pairs, in which the fractured surface follows the helical assembly structure, leading to alternating regions of hills and valleys ( Supplementary Fig. 1 ). These observations also indicate that the helical assembly is right handed, which rotates downwards and clockwise when viewed from the shell’s outer surface ( Fig. 2d ). Corresponding 3D models in Fig. 2a,c show excellent agreement between the proposed structure and experimental observations. Polished transverse cross-sections provide further evidence of the helical assembly of the fibrous building blocks ( Fig. 2e,f ) and multiple series of parabolic arced patterns with alternating transversely (T) and parallel (P) cut regions were observed. Similar patterns have been demonstrated in other well-studied helicoidal structures, which have been found in a variety of natural fibre composites based on cellulose, chitin and collagen [21] , [22] , [23] . The two-dimensional (2D) helicoidal pattern results from transversely cutting a laminate structure in which the orientation of the straight fibres within each lamina is rotated by a small angle with respect to adjacent layers. In the polished C. pyramidata cross-section, the fibre orientations in region P exhibit an oblique angle with respect to the surface by ~20° ( α ), whereas the fibre orientations in a helicoidal structure are always parallel to the surface [21] , [22] , [23] . In fact, α is directly related to the pitch, λ , and diameter, R , of the helix by ( Fig. 2d ). With the experimentally measured value of the helix pitch (~26 μm, as described below in detail), the angle α is estimated to be ~15–22°, consistent with the experimental observations. 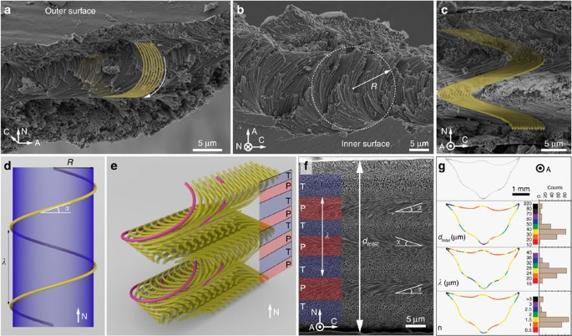Figure 2: Helical assembly of fibrous building blocks. (a) Oblique-, (b) bottom- and (c) cross-sectional-viewed SEM images of fractured surfaces from theC. pyramidatashell, showing the helical assembly with curved fibrous building blocks. Inaandc, the corresponding structures are shown alongside the proposed 3D models. (d) A 3D model that represents the hypothesized helical assembly scheme of curved fibrous building blocks. Note that the curved fibres are not necessarily complete helices through the thickness. Characteristic dimensions of this helical assembly includeR, radius of helix;λ, pitch of helix;α, inclination angle with respect to the horizontal plane. (e) A 3D rendering of the helical assembly with a vertically cut cross-section. Two representative helices are highlighted in purple and the one on the right is partially cut by the cross-sectional plane. P and T are regions where the fibrous building blocks are parallel and transversely cut, respectively. (f) SEM image of a polished cross-section.dtotal, the total thickness of the shell. (g) Mapping dimensional parameters (dtotal,λandn) along the entire shell cross-section (total number of measurements: 204).n, number of periods. From top to bottom, cross-sectional SEM image,dtotal,λandn. The histograms on the right show the statistical distribution of each parameter. N, normal; A, apical; C, circumferential. Figure 2: Helical assembly of fibrous building blocks. ( a ) Oblique-, ( b ) bottom- and ( c ) cross-sectional-viewed SEM images of fractured surfaces from the C. pyramidata shell, showing the helical assembly with curved fibrous building blocks. In a and c , the corresponding structures are shown alongside the proposed 3D models. ( d ) A 3D model that represents the hypothesized helical assembly scheme of curved fibrous building blocks. Note that the curved fibres are not necessarily complete helices through the thickness. Characteristic dimensions of this helical assembly include R , radius of helix; λ , pitch of helix; α , inclination angle with respect to the horizontal plane. ( e ) A 3D rendering of the helical assembly with a vertically cut cross-section. Two representative helices are highlighted in purple and the one on the right is partially cut by the cross-sectional plane. P and T are regions where the fibrous building blocks are parallel and transversely cut, respectively. ( f ) SEM image of a polished cross-section. d total , the total thickness of the shell. ( g ) Mapping dimensional parameters ( d total , λ and n ) along the entire shell cross-section (total number of measurements: 204). n , number of periods. From top to bottom, cross-sectional SEM image, d total , λ and n . The histograms on the right show the statistical distribution of each parameter. N, normal; A, apical; C, circumferential. Full size image We further measured the total thickness ( d total ) and number of periods ( n ) along an entire transverse cross-section of the shell (total number of measurements: 204, Fig. 2g ). Interestingly, the shell maintains the helix pitch ( λ ) within a relatively narrow range (Avg±s.d., 25.5±3.6 μm), while the total shell thickness varies significantly from ~20 to ~200 μm (41.3±26.4 μm). This indicates that the shell’s thickness varies by adjusting the number of periods instead of changing the pitch. Moreover, it is also noted that the shell increases its local thickness at regions with relatively large curvatures (such as the ridges), where stress concentrations are likely generated on loading. Additional structural characteristics of the helical fibrous building blocks were revealed by transmission electron microscopy (TEM) imaging of the cross-sectional samples prepared using focused ion beam milling (FIB, Fig. 3 ). Similar to the cross-sectional scanning electron microscopic (SEM) images, alternating regions with fibres transversely and parallel cut (T and P regions, respectively) were observed ( Fig. 3a,b ). The intersecting angle of the fibres in region P with respect to the shell surface is again ~20°, consistent with the helical structure model. Interestingly, in region T, we observed that the mosaic assembly of the building blocks results from the interlocking of tiles with cross-sectional geometries, such as , and ( Fig. 3b–g ), similar to the structures observed in the shell of the pteropod Cavolinia uncinata [20] . Despite its apparently almost random organization, several key characteristics emerge on close examination. First, the interface boundaries among building blocks are generally parallel or perpendicular to the surface normal (N). This feature is directly correlated to its crystallographic texture, as discussed in the following section. Second, the geometries of these cross-sections are anisotropic. The width of the upper regions (positive N) of the fibres, near the outer shell surface, is ~250 nm (measured along the A direction) and reduces to ca. 100 nm towards the lower portion, resulting in , and shapes ( Supplementary Fig. 2 ). Third, the portions towards the outer shell surface within each cross-section have a high abundance of particle-shaped inclusions with lower average electron density as compared with the surrounding crystalline matrix ( Fig. 3e ). These inclusions are believed to be intracrystalline organic material [24] , [25] , [26] , which will be discussed in detail below. The high concentration of these inclusions in the upper regions of the fibres near the shell outer surface can be also observed from TEM image taken in region P ( Fig. 3h , yellow arrows). 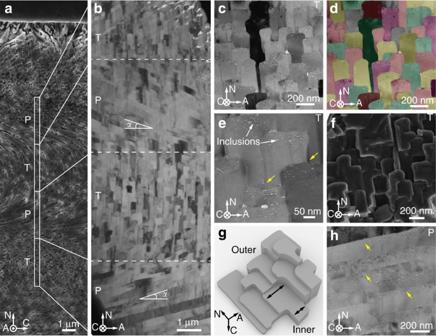Figure 3: Interlocked cross-sections of the helical fibrous building blocks. (a) SEM image of a polished cross-section through aC. pyramidatashell marked with the location and orientation where the TEM sample was prepared using FIB milling (white box); the corresponding TEM image is shown inb. P and T are regions where the fibrous building blocks were parallel and transversely cut, respectively. High-magnification (c–e) TEM and (f) SEM images of the interlocked cross-sections of the fibrous building blocks.dis artificially coloured to further illustrate the mosaic interlocking assembly. The yellow arrows ineindicate the triple junctions of three adjacent building blocks. (g) An artistic 3D illustration of the interlocked cross-sections. (h) TEM image of parallel sections of the fibrous building blocks in region P. Yellow arrows indicate the high density of organic inclusions distributed in the regions towards the direction of outer shell surface. N, normal; A, apical; C, circumferential. Figure 3: Interlocked cross-sections of the helical fibrous building blocks. ( a ) SEM image of a polished cross-section through a C. pyramidata shell marked with the location and orientation where the TEM sample was prepared using FIB milling (white box); the corresponding TEM image is shown in b . P and T are regions where the fibrous building blocks were parallel and transversely cut, respectively. High-magnification ( c – e ) TEM and ( f ) SEM images of the interlocked cross-sections of the fibrous building blocks. d is artificially coloured to further illustrate the mosaic interlocking assembly. The yellow arrows in e indicate the triple junctions of three adjacent building blocks. ( g ) An artistic 3D illustration of the interlocked cross-sections. ( h ) TEM image of parallel sections of the fibrous building blocks in region P. Yellow arrows indicate the high density of organic inclusions distributed in the regions towards the direction of outer shell surface. N, normal; A, apical; C, circumferential. Full size image Crystallographic texture Biomineralized materials are usually highly textured, which has a direct effect on their mechanical properties [27] , [28] , [29] . We investigated the multiscale crystallographic characteristics of the C. pyramidata shell via X-ray and electron diffraction at the mm and μm scales, respectively ( Figs 4 and 5 ). Similar to other pteropods, aragonite is the only mineral phase detected in the shell (PDF #00-041-1475, Supplementary Fig. 3 ). The X-ray diffraction-based texture analysis provided large scale collective crystallographic information, as the X-ray spot size, ~0.3 mm, and penetration depth, ~20–50 μm, were greater than the lateral diameter of the helical assembly and the thickness of the shell, respectively. The as-obtained pole figures of {002}, {012} and {202} are presented in Fig. 4a and the corresponding sample orientation is shown in Fig. 4d . The {002} pole exhibits a highly localized intensity close to the centre of the map, indicating that the c axis of the aragonitic building blocks are aligned roughly perpendicular to the shell surface, similar to many other aragonite-based mollusc shells [27] . Two closely spaced subpeaks with similar intensity contributions, indicated by red and white arrows, are separated from each other by 5–10°. 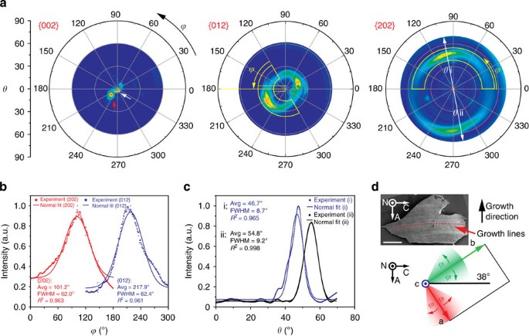Figure 4:Texture analysis of aC. pyramidatashell using X-ray diffraction. (a) Calculated pole density plots for {002}, {012} and {202}. The red and white arrows indicate two subpeaks in the {002} pole figure. (b) Intensity profile versus the azimuthal angleϕintegrated from the yellow sectors in the {012} and {202} pole figures. (c) Intensity profile versus the polar angleθalong the white arrowed line in the {202} pole figure. The corresponding solid lines inbandcare normal fit results. (d) SEM image with sample orientation indicated (top) and the corresponding summarized crystallographic texture. Scale bar ind, 400 μm. FWHM, full width at half maximum; N, normal; A, apical; C, circumferential. Figure 4: Texture analysis of a C. pyramidata shell using X-ray diffraction. ( a ) Calculated pole density plots for {002}, {012} and {202}. The red and white arrows indicate two subpeaks in the {002} pole figure. ( b ) Intensity profile versus the azimuthal angle ϕ integrated from the yellow sectors in the {012} and {202} pole figures. ( c ) Intensity profile versus the polar angle θ along the white arrowed line in the {202} pole figure. The corresponding solid lines in b and c are normal fit results. ( d ) SEM image with sample orientation indicated (top) and the corresponding summarized crystallographic texture. Scale bar in d , 400 μm. FWHM, full width at half maximum; N, normal; A, apical; C, circumferential. 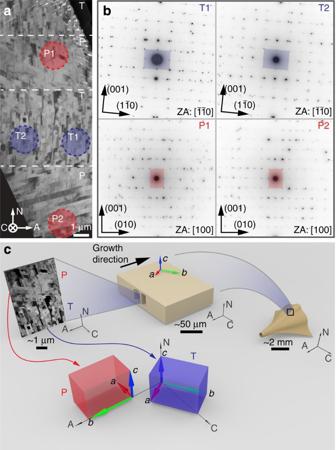Figure 5:Multiscale crystallographic model of theC. pyramidatashell. (a) Cross-sectional TEM image with T and P regions. Four areas labelled as P1, P2, T1 and T2 were used to obtain the selected area electron diffraction (SAED) patterns shown inb. (c) Multiscale crystallographic model inC. pyramidatain relation to the shell geometry based on X-ray diffraction texture analysis and SAED results. N, normal; A, apical; C, circumferential. Full size image Figure 5: Multiscale crystallographic model of the C. pyramidata shell. ( a ) Cross-sectional TEM image with T and P regions. Four areas labelled as P1, P2, T1 and T2 were used to obtain the selected area electron diffraction (SAED) patterns shown in b . ( c ) Multiscale crystallographic model in C. pyramidata in relation to the shell geometry based on X-ray diffraction texture analysis and SAED results. N, normal; A, apical; C, circumferential. Full size image Both {012} and {202} pole figures display a large spread along the azimuthal direction ( ϕ ), which can be quantitatively analysed by integrating the intensity along ϕ (indicated by the yellow sectors, Fig. 4a,b ). The distributions of the two orientations exhibit similar spreads along ϕ as indicated by their similar full width at half maximum with a normal fit ({012}, 62.4°; {202}, 62.0°). The peak positions of the {012} and {202} are located at 217.9° and 101.2°, respectively. This is considered consistent with the theoretical difference of 90° between the two orientations, given the presence of c axis tilt, large in-plane spread and measurement resolution limitations. The full width at half maximum along the polar angle θ for {202} is ~9° ( Fig. 4c ), which is much smaller than the in-plane spread. These results indicate that the shell has a pseudo-fibre-like texture with the aragonite c axis oriented along the surface normal, and with the presence of large in-plane rotations of the a and b axes ( Fig. 4d ). Moreover, the best fit for the b axis is ~38° away from the C direction (calculated by fitting ϕ in the {012} pole figure), that is, the direction of growth lines ( Fig. 4d ). Selected area electron diffraction (SAED) was used to evaluate the local crystallographic information in relation to the corresponding structural features ( Fig. 5 ). The SAED patterns obtained from adjacent transverse and parallel regions indicate that they share similar c axis orientations along the surface normal, although a slight tilt of ~5° was observed in T regions ( Fig. 5a,b ). Moreover, T and P regions do not share the same zone axis, indicating the presence of crystallographic axes rotation along the c axis. In particular, the zone axis of [ ] in region T is in excellent agreement with the crystallographic model based on X-ray diffraction texture analysis. Integrating the information obtained from the X-ray-based texture analysis and SAED measurements, we can construct a multiscale crystallographic model in relation to the shell geometry: (1) the c axis of the aragonitic crystals are generally aligned along the surface normal direction; (2) both the a and b axes are parallel to the shell surface with large in-plane rotations due to the different preferred rotation angles for regions with their fibrous building blocks aligned parallel and perpendicular to the A direction ( Fig. 5c ). Nanoscopic features TEM imaging of aragonitic fibre fragments isolated from the shell showed that the dark regions (corresponding to regions with greater thickness) shift positions from one side to the other or completely disappear along the length of the fibre ( Fig. 6a,b ). These observations suggest that the fibre cross-sectional geometry varies along their long axes. Our proposed 3D model illustrates this feature and the corresponding 2D projection in the inset shows a similar pattern ( Fig. 6c ). The variation in the geometry of fibre cross-sections was further revealed by SEM images of fractured surfaces ( Supplementary Fig. 4 ). 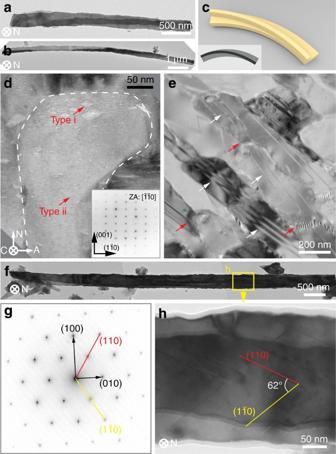Figure 6: Nanoscopic structural features at the building block level. (a,b) TEM images of fragments from isolated individual building blocks. (c) Proposed 3D model of a fibrous building block with axially varying cross-sectional geometry. Inset is the corresponding 2D projection along the N direction showing similar contrast variation as inaandb. (d) TEM image of the cross-section of the building blocks showing the two types (i and ii) of intracrystalline organic inclusions. (e) TEM image of multiple building blocks with twinning bands spanning the entire thickness (white arrows). The red arrows indicate the Moiré fringes. (f) TEM image of an individual isolated building block and (g) its corresponding SAED pattern. (h) TEM image showing the two orientations of twin bands with (110) and () twinning boundaries. N, normal; A, apical; C, circumferential. Figure 6: Nanoscopic structural features at the building block level. ( a , b ) TEM images of fragments from isolated individual building blocks. ( c ) Proposed 3D model of a fibrous building block with axially varying cross-sectional geometry. Inset is the corresponding 2D projection along the N direction showing similar contrast variation as in a and b . ( d ) TEM image of the cross-section of the building blocks showing the two types (i and ii) of intracrystalline organic inclusions. ( e ) TEM image of multiple building blocks with twinning bands spanning the entire thickness (white arrows). The red arrows indicate the Moiré fringes. ( f ) TEM image of an individual isolated building block and ( g ) its corresponding SAED pattern. ( h ) TEM image showing the two orientations of twin bands with (110) and ( ) twinning boundaries. N, normal; A, apical; C, circumferential. Full size image As described earlier, the intracrystalline organic inclusions are heterogeneously distributed within the crystalline fibres, which exhibit relatively high abundance in the upper portions towards the shell outer surface ( Fig. 3c,e,h ). Further examination revealed two types of organic inclusions with different morphologies ( Fig. 6d and Supplementary Fig. 5 ). Type i inclusions, ~20 nm in size ( Supplementary Fig. 6 ), have diamond-shaped projection geometries (viewed at zone axis of [ ], Fig. 6d ), and are typically distributed in upper peripheral regions. Type ii inclusions (thickness, <2 nm) are much more elongated along the basal planes of the aragonite crystals, lack well-defined geometries, and are distributed more homogeneously over an entire building block. (110) twinning bands spanning entire building blocks were observed in cross-sectional TEM images (white arrows, Fig. 6e ). They are typically very thin (width, <5 nm) and the spacing between adjacent twinning bands varies from tens to hundreds of nanometres ( Supplementary Fig. 7 ). TEM imaging and the corresponding SAED patterns of isolated building block fragments revealed multiple twinning bands with multiple crystallographically equivalent twinning boundaries ( Fig. 6f–h ) [30] , [31] . The two twinning boundaries in Fig. 6h form an interplanar angle of 62°, corresponding to the (110) and ( ) twinning boundaries. Moreover, Moiré fringes can be observed along the interfaces between adjacent building blocks (red arrows, Fig. 6e ), which demonstrates the presence of crystallographic misorientations at the building block level. This further contributes to a large in-plane spread of crystal orientations ( Fig. 4 ). Multiscale mechanical behaviour The mechanical behaviour of the C. pyramidata shell was studied via multiple mechanical testing techniques with the aim of understanding the mechanical contribution of the various components of the structural hierarchy across multiple length scales. We first investigated the mechanical significance of the helical assembly by using instrumented microindentation with a sharp cube-corner tip geometry ( Fig. 7a–d ). The maximum loads were varied from 50 to 300 mN, resulting in maximum penetration depths of 4–10 μm, a length scale comparable to the dimensions of the helical assembly. The small displacement bursts of the load-displacement curves ( Fig. 7a ) are corresponding to the microscopic fracture during the indentation tests, as evident by the small fractured pieces near the indentation site ( Fig. 7c ). This phenomenon is similar to the previous observation in another bioceramic shell of Placuna placenta [10] . SEM images of the indents reveal that the indentation residue sites were absent of radial cracks, even when the indentation corner was aligned with the axial direction of the fibrous building blocks ( Fig. 7b,c ). The corresponding optical image clearly reveals the underlying isotropic damage zone without any radial fractures ( Fig. 7d ). The rotating fibrous building blocks in the helical assembly effectively restricted the initiation and propagation of cracks, even when the fibre orientation at the surface was parallel to the side of the cube-corner indenter. These results indicate that the helical structure is able to channel the cracks and damage along the rotating direction of the helical fibrous building blocks, through which the damage can be localized, suppressed and contained within the isotropic damage zone. The propagation of cracks along the helical interfaces between building blocks can be further illustrated by observing the tortuous fracture pattern in naturally damaged shells ( Fig. 7e,f ). 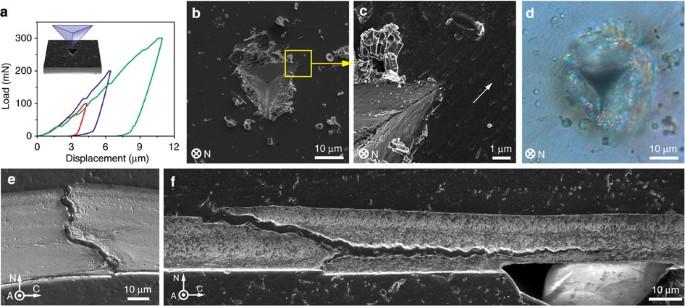Figure 7:Mechanical behaviour of the helical assembly. (a) Representative load–depth curves from the instrumented microindentation experiments with a cube-corner probe on aC. pyramidatashell (maximum loads, 100, 200 and 300 mN). Inset, schematic diagram of the indentation experiment. (b,c) SEM images of the indentation residue, showing the local damage (maximum load, 300 mN). (c) SEM image showing the absence of radial cracks when the indentation corner is aligned with the axial direction of the fibrous building blocks (arrow). (d) The corresponding optical image of the same indentation residue showing the underlying isotropic and circular damage zone. (e) Backscattered SEM image displaying the curved pathway of a naturally formed crack. (f) SEM image of a naturally formed crack constrained within the shell. Figure 7e demonstrates that the crack front followed the helical pattern when penetrating the shell. Figure 7f shows that the crack was channelled within the shell almost horizontally, which avoids catastrophic failure of the shell with a thickness of only ~20 μm. Figure 7: Mechanical behaviour of the helical assembly . ( a ) Representative load–depth curves from the instrumented microindentation experiments with a cube-corner probe on a C. pyramidata shell (maximum loads, 100, 200 and 300 mN). Inset, schematic diagram of the indentation experiment. ( b , c ) SEM images of the indentation residue, showing the local damage (maximum load, 300 mN). ( c ) SEM image showing the absence of radial cracks when the indentation corner is aligned with the axial direction of the fibrous building blocks (arrow). ( d ) The corresponding optical image of the same indentation residue showing the underlying isotropic and circular damage zone. ( e ) Backscattered SEM image displaying the curved pathway of a naturally formed crack. ( f ) SEM image of a naturally formed crack constrained within the shell. Full size image We also explored the smaller length scale mechanical behaviour of the interlocked fibrous building blocks through uniaxial compression of micropillars prepared from C. pyramidata shells using FIB milling ( Fig. 8 ). The average diameter and height of the micropillars were 2.0 and 6.6 μm, respectively ( Fig. 8a,c ). As the diameters of these micropillars were much smaller than the helix diameter, this technique only probed the mechanical response of a few interlocking building blocks. The micropillars were compressed parallel to the shell’s surface normal and the representative force-displacement curves shown in Fig. 8b indicate stepwise damage, in contrast to catastrophic fracture of most brittle ceramic materials. The interlocking microstructure retards the propagation of initial primary cracks and facilitates microcracking, which assures a high density of microcracking and results the generation of multiple tiny fractured pieces during a compression test ( Fig. 8d ). 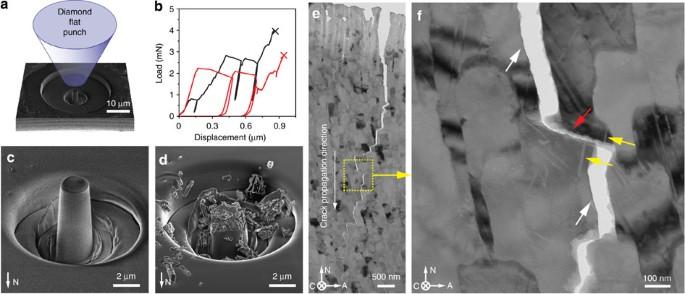Figure 8:Mechanical behaviour of interlocked building blocks. (a) Schematic illustration of the uniaxial compression of microscale pillars. (b) Representative load-displacement curves from micro-compression tests. SEM images of the micropillar (c) before and (d) after compression (tilted at 52°). (e) TEM image showing crack deflection by the microscopic interlocking building blocks. (f) A high-magnification TEM image of a region inedemonstrating different modes of fracture: intergranular fracture (white arrows) and intragranular fracture (red arrow). The crack cut through the (110) twinning boundaries (yellow arrows). N, normal; A, apical; C, circumferential. Figure 8: Mechanical behaviour of interlocked building blocks . ( a ) Schematic illustration of the uniaxial compression of microscale pillars. ( b ) Representative load-displacement curves from micro-compression tests. SEM images of the micropillar ( c ) before and ( d ) after compression (tilted at 52°). ( e ) TEM image showing crack deflection by the microscopic interlocking building blocks. ( f ) A high-magnification TEM image of a region in e demonstrating different modes of fracture: intergranular fracture (white arrows) and intragranular fracture (red arrow). The crack cut through the (110) twinning boundaries (yellow arrows). N, normal; A, apical; C, circumferential. Full size image To further investigate the interaction between crack propagation and the interlocking microstructure, we purposely induced cracking in a TEM sample by fracturing it with a micromanipulator inside an SEM ( Fig. 8e,f ). Subsequent TEM imaging showed that the crack propagated in a tortuous manner at the nanoscale by following the interlocking boundaries between the constituent building blocks ( Fig. 8e ). Clearly, intergranular fracture was the dominant mode of crack propagation, as the crack mainly followed interface boundaries ( Fig. 8f , white arrows). To a lesser extent, intragranular fracture was also observed ( Fig. 8f , red arrow), generating a higher degree of roughness at the nanometre scale relative to intergranular fracture. Interestingly, intragranular fracture generally occurred in the upper regions of the building blocks. The high abundance of intracrystalline organic inclusions in that region might facilitate intragranular fracture, as it has been proposed previously that the presence of organic inclusions in nacre could lead to heterogeneous mechanical properties at the building block level [32] . By controlling the distribution of intracrystalline organic inclusions within individual building blocks, molluscs like C. pyramidata can engineer heterogeneous mechanical properties at the nanoscale, which could lead to enhanced energy dissipation on deformation [6] . Observations of much rougher fractured surfaces in regions of intragranular fracture support this hypothesis ( Fig. 8f and Supplementary Fig. 8 ). Here we should note that the above observations are based on the crack propagation in a 2D TEM sample, where the interfaces between the building blocks were mostly through thickness (<100 nm). Although intergranular and intragranular fracture should both occur in the bulk 3D samples, we believe the latter should be more prevalent due to geometric constraints created by the interlocking building blocks. This hypothesis is further supported by the observation of multiple tiny fractured pieces created during the micropillar compression studies ( Fig. 8d ). Last, the presence of (110) twinning boundaries within the building blocks could potentially also increase resistance to intragranular fracture ( Fig. 8f , yellow arrows). In this work, we present a comprehensive study of the multiscale structural and crystallographic features of the aragonitic shell of the pteropod C. pyramidata . The helical assembly of fibrous building blocks with interlocking cross-sections is one of the most distinctive characteristics of this structure compared with other known calcium carbonate-based molluscan shell microstructures [33] . The pitch and diameter of the right-handed helix consisting of fibrous building blocks are roughly maintained throughout the shell, while the number of periods varies proportionally with the shell thickness. The cross-sectional geometry of each fibre exhibits local variation along their axial directions, a design strategy which has a direct effect on the shell’s structural integrity by creating a 3D interlocking architecture. The non-uniform cross-section of each building block is also geometrically necessary to produce a closely packed composite, as it is impossible to build a composite structure in which adjacent helical fibres with uniform cross-sectional geometries are uniformly spaced with respect to each other [34] . This so-called isomorphic packing of helical fibres inevitably generates uneven spacing between the fibres, leading to the formation of voids [34] . It is experimentally challenging to determine whether the fibres in the helical assembly are continuous through the entire thickness of the shell, although the crystallographic analysis suggests that they are not. Large in-plane rotation of a and b axes with respect to the shell surface normal (that is, c axis) suggests the possibility of crystallographic discontinuities through the thickness, which was confirmed by local SAED measurements. With the reasonable assumption that each building block is a single crystalline [35] , [36] (also supported by electron diffraction results of individual isolated fibres, Fig. 6g,h ), we hypothesize that the fibres most likely do not exhibit a complete helical form. Instead, through the thickness of the shell (N direction), regions with curved fibrous building blocks with preferred a and b axes distributions are stacked together along N to complete the helical assembly, while always maintaining the c axis oriented normal relative to the shell surface. With the multiscale mechanical testing methods, we found that the C. pyramidata shell exhibits exceptional fracture resistance due to its complex hierarchical design. At the macroscopic level (mm–cm), the pyramidally shaped shell is thickened at the sharp corners by increasing the number of helical periods, which enhances the resistance to damage initiation at these locations of stress concentration. At the microscopic level (~10–100 μm), the unique helical organization of the fibrous building blocks distinguishes itself from other mineralized mollusc microstructure types [33] , even when compared with fibre-based biological materials with higher organic contents [21] , [22] , [23] . As revealed by both microindentation experiments and naturally damaged shells, cracks tend to follow along the helical interfaces of the fibres, which rotate and nest volumetrically within the shell, hindering the catastrophic propagation of cracks through the shell thickness. This behaviour leads to the generation of a much larger surface area per unit crack length in the thickness direction, amplifying energy dissipation during deformation. The toughening mechanism achieved through the generation of a tortuous crack trajectory is very similar to that observed in both biological and engineering plywood composite materials [23] . However, two important unique and advantageous features of this helical assembly should be noted. First, the variation of the cross-sectional geometry of the fibres along the axial directions promotes crack deflection at the nanoscale (and discussed in detail below), further increasing resistance to crack propagation. Second, simple plywood composite materials suffer delamination failure through the weak in-plane interfaces [5] , [37] , which results in low resistance against out-of-plane impact [38] . The helical organization of fibrous building blocks can potentially minimize this problem by having 3D interfaces without the presence of large in-plane weak interfaces where delamination might occur. Moreover, the helical assembly is also able to achieve greater mechanical isotropy, which is desired for in-plane loading and achieved in engineering laminate composites by stacking laminae with different orientations. Thanks to the continuous rotation of the fibre orientation through the thickness, the shell is able to isotropically constrain damage without forming large radial cracks even when the axial direction of the fibres is aligned with the corner of the microindenter tip. At the nano/microscopic level (~0.5–10 μm), the interlocking cross-sections of the fibrous building blocks lead to crack deflection along the interfaces between them, which acts as a toughening mechanism operating at crack tips. This process follows the well-known Cook–Gordon mechanism for crack deflection with the presence of weak interfaces ahead of the crack tip [39] . Moreover, unlike most metal and ceramic engineering polycrystalline materials with pseudo-hexagonal grains, the cross-sections in C. pyramidata have triple junction grain angles close to 90° (as compared with ~120° in engineering materials) and concave boundaries (the inner angles are >180°). Compared with pseudo-hexagonal grains, the 90° triple junctions can greatly reduce the local mode I stress intensity factor ( k 1 ) by orthogonally deflecting a primary crack [40] . The interlocking effect produced from concave grain boundaries further restricts the propagation of cracks. Engineering the grain microstructure in terms of size, shape and distribution has already been shown to enhance the strength and fracture toughness of engineering metals and ceramics [41] , [42] , [43] , although few synthetic materials can currently match biological materials in terms of structural control at nano/microscopic length scales. At the macroscopic level, however, the design of structural materials with interlocking building blocks has recently been successfully demonstrated to enhance the fracture resistance and damage tolerance [18] , [19] . Last, the anisotropic cross-sectional shape of the building blocks with larger widths in their upper regions lead to a higher degree of crack deflection as the crack tip can ‘explore’ multiple directions at the bifurcating grain junctions. At the nanoscopic level (~1–500 nm), structural features within individual building blocks start to play a role in enhancing fracture resistance. It has been hypothesized that the presence of intracrystalline organic inclusions improve mechanical performance and are responsible for the conchoidal fracture surfaces often observed in biominerals [44] , [45] . Here we provide evidence that the heterogeneous distribution of intracrystalline organic components is likely able to promote intragranular fracture, leading to rough fractured surfaces at the nanoscale. This phenomenon is not likely limited to this system, as heterogeneous distributions of organic inclusions have been observed in several other biomineralized structures [46] , [47] . The nanoscale compositional heterogeneity leads to mechanical property variation at the same length scale, which further enhances energy dissipation [6] . Moreover, the presence of {110} twinning boundaries likely provides further resistance to damage by constraining dislocation motion and deflecting cracks [10] , [48] . In addition to the geometrical and structural characteristics discussed above, the unique crystallographic texture also contributes to the mechanical robustness. First, the fibre-like texture with the c axis oriented along the surface normal provides greater hardness and stiffness due to the anisotropic mechanical properties of aragonite [49] . While maintaining the out-of-plane anisotropy, the in-plane mechanical isotropy is enhanced through the large in-plane rotation of the crystallographic directions in the helical assembly. Moreover, the crystallographic misorientations at the building block level lead to mechanical heterogeneity through crystallographic rather than compositional control, which might lead to the enhanced energy dissipation at the nanoscale [6] . The mechanisms discussed above at different length scales work synergistically to enhance the fracture resistance and damage tolerance of the shell of the pteropod C. pyramidata . This allows the shell to be mechanically robust even though it is extremely thin (~40 μm) and lightweight (~13 mg), which is critically important for this pelagic gastropod. Moreover, another benefit of an ultrathin shell is its extremely high light transmission capability (up to ~80% at wavelength of 600 nm, Supplementary Fig. 9 ). Optical transparency as a camouflage strategy for anti-predation has been found in a variety of terrestrial, freshwater and marine organisms, including some pelagic pterotracheid and carinariid heteropods, pseudothecosomatous pteropods, and phylliroid nudibranchs [50] , [51] , [52] . Therefore, we hypothesize that, similar to other non-shelled pteropods, the camouflage strategy through transparency might also be utilized as a self-protection mechanism for this shelled species. The intricate structural and crystallographic design of this protective shell is the evolutionary result of multiple selective pressures, including but not limited to mechanical protection, locomotion and transparency camouflage. The detailed multiscale materials design principles for the fracture resistance discovered here might therefore provide effective guidelines and strategies for the development of advanced engineering (transparent) structural materials. Samples Dried C. pyramidata shells were kindly provided by Smithsonian National Museum of Natural History (Washington DC, USA). The aperture region of these shells was damaged during sample collection ( Fig. 1a,b ), which was likely due to bending deformations along the growth margin. Micro-CT The complete shells of C. pyramidata were scanned via synchrotron X-ray microtomography (15 keV) at beamline 2BM at the Advanced Photon Source of Argonne National Laboratory (Chicago, USA). The resulting X-ray projection images of the scanned sample were converted into 3D polygonal meshes (stereo-lithography, STL) using an interactive medical image processing system (MIMICS 9.0, Materialise, Belgium) and rendered using the computer-aided design software, Blender. Electron microscopy Fractured or polished shell samples were carbon coated to reduce charging effects before SEM imaging with a Helios Nanolab 600 Dual Beam (FEI, OR) at an acceleration voltage of 2 kV and working distance of 4 mm. TEM samples were prepared using the same system. A detailed TEM sample preparation procedure is as follows: (1) a platinum protective layer (~0.5 μm) was first laid down on top of the desired region; (2) another platinum protective layer (~1.5 μm) was further deposited on top of the region where the slab was to be milled out; (3) two trenches, one on each side of the platinum protective stripe, were milled by FIB, leaving the specimen slab (thickness: ~1.5 μm); (4) the slab was then cut through by FIB and transferred to a copper TEM grid by an Omniprobe and welded securely via platinum deposition; (5) the lift out lamellar specimen was sequentially thinned by FIB at 30, 16, 5 and 2 kV ion beam voltages. Final polishing at 2 kV, 28 pA was critical for obtaining a clean surface with minimum amounts of damage. TEM imaging with typical bright-field, dark-field and SAED techniques was carried out using a JEOL 2011 TEM operated at 120 kV. The image magnification and camera constants were calibrated using a standard sample (MAG*I*CAL, Electron Microscopy Sciences, PA, USA). The high resolution TEM imaging was performed on a JEOL 2010F operated at 200 kV. Whole-shell SEM imaging was performed with a Tescan Vega SEM. 3D reconstruction of the fracture surfaces was achieved by first taking stereo SEM image pairs with the sample stage tilted at 10° and −10°, and then analysing and rendering with MountainsMap SEM imaging analysis software. X-ray diffraction A piece of shell was fractured (~2 mm) and fixed on a silicon wafer substrate using adhesives. The crystallographic pole figures were obtained using a Bruker D8 diffractometer (Cu Kα radiation with a wavelength of 1.5406 Å) with the General Area Detector Diffraction System (GADDS, equipped with a Vantec2000 2D detector). The incident X-ray beam was conditioned with an incident beam graphite monochromator and a monocapillary lens. The size of the X-ray spot was estimated to be ~0.3 mm in diameter and the penetration depth was ~20–50 μm. After the diffraction measurement, the sample was imaged using a Helios Nanolab 600 Dual Beam (FEI, OR). Microindentation Microindentation experiments were carried out on the C. pyramidata shell with a Micro Materials microindenter (Wrexham, UK) in ambient conditions. Load-controlled indentation was performed using a sharp cube-corner diamond tip. Typical load functions include loading (30 s), holding (5 s) and unloading (30 s). The maximum load was varied from 50 to 300 mN. Sample drifting was monitored when the force was unloaded to 5% of the maximum force for 40 s. Uniaxial micropillar compression Micropillars were prepared via FIB milling with a Helios Nanolab 600 Dual Beam (FEI, OR). A top–down annular milling technique was applied at 30 kV accelerating voltage with the current decreased stepwise from 9.3 nA to 48 pA. The diameter of the outer trench around the pillar was 30 μm to provide clearance for the compression test. The diameter and height of the as-prepared micropillars were 1.5–2.5 μm and 5–8 μm, respectively. The micro-compression experiments were carried out on a Hysitron Triboindenter with a flat punch diamond tip (tip diameter: 10 μm) under displacement control (displacement rate: 40 nm s −1 ). How to cite this article: Li, L. et al . Hierarchical structural design for fracture resistance in the shell of the pteropod Clio pyramidata . Nat. Commun. 6:6216 doi: 10.1038/ncomms7216 (2015).